Sansanmycin natural product analogues as potent and selective anti-mycobacterials that inhibit lipid I biosynthesis Tuberculosis (TB) is responsible for enormous global morbidity and mortality, and current treatment regimens rely on the use of drugs that have been in use for more than 40 years. Owing to widespread resistance to these therapies, new drugs are desperately needed to control the TB disease burden. Herein, we describe the rapid synthesis of analogues of the sansanmycin uridylpeptide natural products that represent promising new TB drug leads. The compounds exhibit potent and selective inhibition of Mycobacterium tuberculosis , the etiological agent of TB, both in vitro and intracellularly. The natural product analogues are nanomolar inhibitors of Mtb phospho-MurNAc-pentapeptide translocase, the enzyme responsible for the synthesis of lipid I in mycobacteria. This work lays the foundation for the development of uridylpeptide natural product analogues as new TB drug candidates that operate through the inhibition of peptidoglycan biosynthesis. Tuberculosis (TB) is caused by infection with the bacterium Mycobacterium tuberculosis ( Mtb ) and, according to the World Health Organization, was responsible for 1.5 million deaths and the emergence of 9.6 million new cases of the disease in 2014 (ref. 1 ). Current treatment for TB relies on a 6-month quadruple therapy comprising rifampicin, isoniazid, ethambutol and pyrazinamide [2] . Despite achieving a cure rate of >95% for drug-sensitive TB, this regimen is not effective against multi-drug resistant (MDR) and extensively drug resistant (XDR) TB infections, which are emerging at an alarming rate globally. While MDR infections can be treated with second-line antibiotics for extended periods, XDR infections are virtually untreatable as exemplified by a 98% mortality rate in a recent outbreak in South Africa [3] . To effectively combat these drug resistant cases, new TB drugs with novel modes of action are desperately needed. Two compounds, bedaquiline and delamanid, were recently approved for drug resistant TB; however these are only used as drugs of last resort owing to reported toxicity issues [4] . It is well established that natural products provide a rich resource for the discovery of new drug leads [5] , [6] . Approximately 65% of antibacterials approved for use between 1981 and 2010 were natural products or natural product derivatives [5] , [6] , including currently employed TB drugs for example, rifampicin and the aminoglycosides. The sansanmycins belong to the uridylpeptide natural product family, a sub-class of the structurally diverse nucleoside antibiotics [7] , [8] that include the liposidomycins [9] , caprazamycins [10] , capuramycins [11] , [12] and muraymycins [13] . The sansanmycins are produced by the soil bacterium Streptomyces sp. [14] , [15] , [16] and have a number of interesting structural features that are unique to the uridylpeptide natural product family. These include a 3′-deoxyuridine motif appended to N -methyl-2,3-diaminobutyric acid (DABA) via an unusual cis -4′,5′-enamide linkage. The DABA moiety is found within a ‘ pseudo -tetrapeptide’ chain which possesses the sites of variation in the family [7] . In addition to these fascinating structural features, the natural products have been shown to possess significant activity against Mtb , including MDR strains [14] , [15] . For these reasons we became interested in the sansanmycin scaffold as a privileged starting point for the discovery of novel TB drug leads. In this manuscript we describe the rapid synthesis of a library of sansanmycin analogues that exhibit potent and selective activity against the virulent H37Rv strain of Mtb . We show that these natural product analogues disrupt the activity of Mtb phospho-MurNAc-pentapeptide translocase (variously designated as MurX in mycobacteria, MraY or translocase I in the literature), the integral membrane enzyme responsible for the biosynthesis of lipid I, a key intermediate in mycobacterial peptidoglycan synthesis. Anti-mycobacterial activity of dihydrosansanmycin A–C Our initial goal focused on gaining access to structural analogues of the sansanmycin uridylpeptide natural product family (for example, analogues of sansanmycin A–C 1–3 (refs 14 , 15 ), Fig. 1 ). To date, several derivatives of uridylpeptide natural products have been generated through engineering of the organisms that produce the natural products or through semi-synthetic approaches and, as such, feature limited structural variation [17] , [18] , [19] , [20] , [21] , [22] , [23] , [24] , [25] . A number of synthetic studies have also been reported on uridylpeptide natural products and analogues [26] , [27] , [28] , [29] , [30] , [31] , [32] , [33] , some of which have been shown to possess antimicrobial activity [7] , [8] . The focus of the present study was to develop a rapid and divergent synthetic strategy to access a diverse library of sansanmycin analogues that would enable the determination of key structure-activity relationships specifically against Mtb. In previous studies it has been shown that dihydropacidamycin analogues, lacking the enamide linkage maintained activity against Pseudomonas aeruginosa [23] . Given the potential metabolic lability of the enamide, we chose to target dihydrosansanmycin analogues in this study. Following the preparation of the first targets ( Supplementary Methods ) dihydrosansanmycins A–C ( 4 – 6 ), screening against the virulent H37Rv strain of Mtb was conducted using a resazurin assay [34] ( Fig. 1 ). These compounds were also counter-screened against HEK293 cells to gauge selectivity ( Supplementary Methods ). We were pleased to find that sansanmycin analogues 4–6 exhibited significant inhibitory activity against Mtb , with dihydrosansanmycin A ( 4 ) and B ( 5 ) possessing nanomolar MIC 50 values ( Fig. 1 ). Crucially, the stereochemistry at C-4′ of the ribose moiety was shown to be essential for anti-mycobacterial activity, with S -configuration in a dihydrosansanmycin B analogue leading to complete loss of activity ( Supplementary Fig. 30 ). Interestingly, the importance of stereochemistry at C-4′ has also been reported for dihydropacidamycin, whereby analogues with S -stereochemistry at this position exhibited reduced activity against P. aeruginosa compared with the corresponding R -epimer [23] . 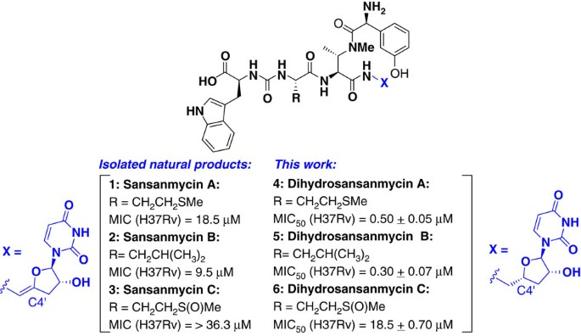Figure 1: Structures of sansanmycins A-C (1–3), synthetic dihydrosansanmycins A–C (4–6) and inhibitory activity againstMtbH37Rv. MIC values of isolated sansanmycins A–C (1–3) were previously reported by Xieet al.14,15MIC50values of4–6represent the average of two independent experiments, each performed in triplicate; positive controls RIF: MIC50=0.006±0.002 μM; INH: MIC50=0.025±0.005 μM; MIC50(HEK293) for4–6>200 μM. Figure 1: Structures of sansanmycins A-C (1–3), synthetic dihydrosansanmycins A–C (4–6) and inhibitory activity against Mtb H37Rv. MIC values of isolated sansanmycins A–C ( 1–3 ) were previously reported by Xie et al . [14] , [15] MIC 50 values of 4–6 represent the average of two independent experiments, each performed in triplicate; positive controls RIF: MIC 50 =0.006±0.002 μM; INH: MIC 50 =0.025±0.005 μM; MIC 50 (HEK293) for 4–6 >200 μM. Full size image Synthesis and activity of dihydrosansanmycin analogues Encouraged by the promising anti-mycobacterial activity of dihydrosansanmycin B ( 5 ), we next focused on the preparation of a targeted library of analogues of 5 to delineate the functional importance of the non-proteinogenic amino acid m -tyrosine ( m -Tyr). As such, analogues 7–17 , retaining the DABA unit (due to the previously established importance of the N - and β-methyl moieties for activity [28] , [32] , [33] ) but possessing a variety of functionalities in place of the m -Tyr moiety, were proposed ( Fig. 2 ). Here, we took the opportunity to develop a robust divergent route to rapidly access the analogues. Preparation of 7–17 began with the synthesis of fully protected isopeptide fragments via Fmoc-strategy solid-phase peptide synthesis on 2-Cl Trt Cl resin. This was followed by late stage coupling of 4′-deoxyuridine fragment 18 which was synthesized from uridine in 12 steps using modifications to a method reported by Boojamra et al . [23] ( Fig. 2 , Supplementary Methods ). Two approaches were employed to access members of the library. The first involved coupling of suitably protected preformed isopeptide building blocks with a variety of amino acids appended to the DABA unit (general structure 19 ). The second strategy involved the installation of allyloxycarbonyl (Alloc)-protected DABA fragment 20 onto the solid phase. This enabled late stage divergent access to the desired pseudo peptidic structures through en bloc Pd(0) deprotection followed by coupling of a variety of amino acids (R 1 in Fig. 2 , Supplementary Methods ). 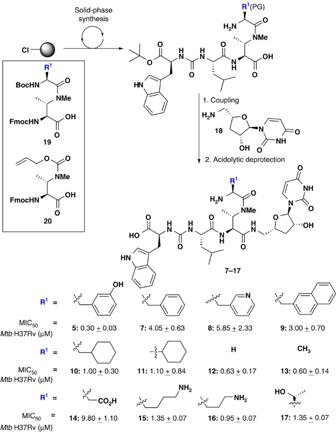Figure 2: Synthesis of 1st generation sansanmycin analogues 7–17 with inhibitory activities againstMtbH37Rv. PG=side chain protection necessary for the synthesis of5,14,15and16. MIC50values represent an average of two independent experiments each performed in triplicate; positive controls RIF: 0.006±0.002 μM; INH: MIC50=0.025±0.005 μM; MIC50(HEK293) for7–17>200 μM. Figure 2: Synthesis of 1st generation sansanmycin analogues 7–17 with inhibitory activities against Mtb H37Rv. PG=side chain protection necessary for the synthesis of 5 , 14 , 15 and 16 . MIC 50 values represent an average of two independent experiments each performed in triplicate; positive controls RIF: 0.006±0.002 μM; INH: MIC 50 =0.025±0.005 μM; MIC 50 (HEK293) for 7–17 >200 μM. Full size image Following synthesis and purification by reverse-phase HPLC, analogues 7–17 were assessed against Mtb (H37Rv). We were pleased to find that most of the analogues retained significant activity against Mtb , albeit with a relatively flat structure-activity profile, with MIC 50 values ranging from 0.6 to 9.80 μM for the series ( Fig. 2 ). The incorporation of alternative aromatic substituents in compounds 7–9 proved to be detrimental with over an order of magnitude drop in activity. Incorporation of cyclohexyl-Ala ( 10 ), cyclohexyl Gly ( 11 ), Lys ( 15 ), Orn ( 16 ) or Thr ( 17 ) residues in place of m -Tyr did not lead to an appreciable decrease in activity (MIC 50 =0.95–1.35 μM), with the exception of the negatively charged Asp residue in 14 which led to a significant drop in potency. Interestingly, the replacement of m -Tyr with amino acids with smaller side chains for example, Gly in 12 (MIC 50 =0.63 μM) and Ala in 13 (MIC 50 =0.60 μM), provided anti-mycobacterials that were more potent than other substitutions at this position. As with dihydrosansanmycin A–C ( 4–6 ), compounds 7–17 were not cytotoxic to HEK293 cells up to a concentration of 200 μM. Given the promising activity of the natural product analogues against Mtb , we were next interested to assess the antimicrobial activity against other pathogenic bacteria to gauge whether there was any selectivity in activity. Towards this end, we counter-screened 4–17 against a panel of 15 pathogenic Gram-negative and Gram-positive bacterial strains using a high throughput screen, including several ‘ESKAPE’ pathogens of clinical relevance [35] . The organisms in the screen included: Bacillus subtilis , Staphylococcus aureus, methicillin-resistant S. aureus (MRSA), Staphylococcus epidermidis, Listeria ivanovii, Enterococcus faecium , Escherichia coli, Vibrio cholerae, Salmonella typhimurium, Pseudomonas aeruginosa, Yersinia pseudotuberculosis, Providencia alcalifaciens, Ochrobactrum anthropi, Enterobacter aerogenes, Acinetobacter baumannii . Remarkably, while a small number of compounds exhibited modest activity against E. coli and P. aeruginosa (MIC 50 s: 12.5–100 μM), most did not inhibit the growth of other strains up to concentrations of 100 μM ( Supplementary Tables 1 and 2 ). This selective anti-mycobacterial activity is an important criterion for the development of a TB drug lead and, as such, was a particularly encouraging observation. Second-generation dihydrosansanmycin analogues Because substitution of the synthetically challenging m -Tyr residue in 5 with a Gly residue in 12 did not lead to a substantial drop in anti-mycobacterial activity, we chose to maintain Gly at this position, and modify the Leu residue within the peptide chain (R in Fig. 1 ), in a second generation compound library. Specifically, a number of alkyl, heteroalkyl, aryl and heteroaryl substituents were proposed in analogues 21–36 with a view to interrogating further SARs. Dihydrosansanmycin analogues 21–36 were synthesized using the divergent solid-phase strategy described above ( Supplementary Methods ) and assessed for anti-mycobacterial activity against Mtb H37Rv ( Fig. 3 ). Substitution of the isopropyl sidechain in 12 with different alkyl side chains in 21–24 did not lead to substantial differences in activity with MIC 50 values ranging from 510 to 930 nM. Interestingly, extension of the cyclohexyl Gly side chain in 24 with a cyclohexyl Ala moiety led to a substantial increase in potency with analogue 25 exhibiting an MIC 50 of 80 nM against Mtb . The introduction of more polar substituents, for example, a Thr side chain in 26 or an Asp residue in 27 led to a significant drop in activity (MIC 50 =2.80 μM and >6.25 μM, respectively) when compared with original lead 12 . A similar drop in activity was not observed when a Lys residue was introduced in 28 which was equipotent to 12 (MIC 50 =700 nM). Incorporation of aryl and heteroaryl groups in 29–36 in place of the Leu residue in 12 generally gave rise to improved anti-mycobacterial activity. Indeed, introduction of a Phe residue in 29 or a p -CF 3 Phe residue in 30 led to a two-fold improvement in activity compared with 12 . Substitution with Tyr ( 31 ), 3-pyridyl Ala ( 32 ) and Trp ( 33 ) residues led to a modest drop in activity against Mtb compared with 29 (MIC 50 =0.44–0.98 μM). Shortening the side chain of Phe derivative 29 with a phenyl Gly side chain in 34 resulted in a dramatic drop in activity (MIC 50 >6.25 μM). This is in line with the reduced activity observed when shortening the side chain in the homologous analogues 24 and 25 with saturated cyclohexyl functionalities. Extending the Phe side chain in 29 by a further methylene unit in homo-Phe derivative 35 led to a four-fold loss in activity, while the incorporation of a naphthyl Ala side chain in 36 provided the most potent compound in the aryl substituted series with an MIC 50 of 180 nM against Mtb . As with the first generation series of dihydrosansanmycin analogues, 21–36 did not show any activity (up to 200 μM) against HEK293 cells, and exhibited poor or no activity against the 15 pathogenic Gram-positive and Gram-negative bacterial strains ( Supplementary Tables 1 and 2 ). 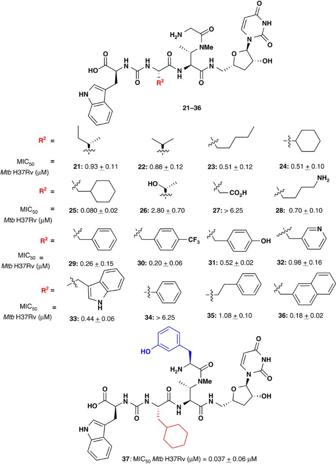Figure 3: Synthesis of 2nd generation sansanmycin analogues 21–37 with inhibitory activities againstMtbH37Rv. MIC50values represent average of two independent experiments, each performed in triplicate; positive controls RIF: MIC50=0.006±0.002 μM; INH: MIC50=0.025±0.005 μM; MIC50(HEK293) for21–37>200 μM. Figure 3: Synthesis of 2nd generation sansanmycin analogues 21–37 with inhibitory activities against Mtb H37Rv. MIC 50 values represent average of two independent experiments, each performed in triplicate; positive controls RIF: MIC 50 =0.006±0.002 μM; INH: MIC 50 =0.025±0.005 μM; MIC 50 (HEK293) for 21–37 >200 μM. Full size image On the basis of the first generation ( 7–17 , Fig. 2 ) analogue library, the optimal isopeptide substitution on the DABA unit was m -Tyr (found natively in the sansanmycins), whilst in the second generation library ( 21–36 , Fig. 3 ), a cyclohexyl Ala residue provided the most potent anti-mycobacterial activity. With this in mind, analogue 37 was designed and synthesized that incorporated both of these functionalities ( Fig. 3 , Supplementary Methods ). Gratifyingly, this analogue possessed the most potent activity against Mtb of all the natural product analogues synthesized with an MIC 50 of 37 nM. Mechanism of action of sansanmycin analogues It has been hypothesized that the antibacterial mechanism of action of the nucleoside antibiotic family is via inhibition of translocase I (MraY), an integral membrane protein that transfers UDP-MurNAc pentapeptide to polyisoprenylphosphate phosphate to afford lipid I, thereby catalysing the first membrane-associated step of peptidoglycan biosynthesis ( Fig. 4a ) [7] . Whilst inhibition of MraY has been unequivocally determined for some members of the family [8] , [25] , [28] , [36] , [37] , [38] , including a recently published structure of a complex of muraymycin D2 with the Aquifex aeolicus enzyme [25] , the antibacterial activity of other nucleoside antibiotics, including the sansanmycins, have only been predicted to be caused by inhibition of this enzyme. Furthermore, structural analogues of the nucleoside antibiotics have, on several occasions, been shown not to inhibit MraY, but to target other essential enzymes, suggesting that structural changes to the natural product can attenuate and even switch activity to other bacterial enzymes [39] , [40] . We were therefore interested in assessing the inhibitory activity of dihydrosansanmycin analogues 7–17 and 21–37 against Mtb translocase I. It is important to note that while the translocase I enzyme is dubbed MraY in most organisms, in mycobacteria this enzyme is encoded by the murX gene and is therefore referred to as MurX. An assay was developed to assess the inhibitory activity of the natural product analogues against Mtb MurX in an initial screen. Consistent with prior work on MraY orthologues of Mtb MurX (ref. 41 ), we were unable to overexpress the enzyme and therefore opted to assay the native enzyme in mycobacterial membranes. Briefly, Mtb mc 2 6230 membrane protein preparations were generated that contained MurX, along with other membrane proteins (including MurG, the enzyme that generates lipid II from lipid I, Fig. 4a ). The inhibition of MurX was assessed in a MurX–MurG coupled assay whereby a decrease in lipid II formation was monitored by radiochemical means. Because the nucleoside antibiotics have only been demonstrated to inhibit MurX, we made the assumption that, despite the coupled nature of the assay, it would serve to effectively measure the inhibition of MurX. The assay was initially performed by the addition of a 200 nM concentration of a given sansanmycin analogue together with UDP-[ 14 C]GlcNAc and UDP-MurNAc pentapeptide (Park’s nucleotide). Following quenching of the enzymatic reactions and an extraction-based work up, thin layer chromatography (TLC) and phosphorimaging were used to measure the degree of inhibition of MurX by measuring a decrease in the formation of lipid II that incorporated the [ 14 C] label on the GlcNAc moiety ( Fig. 4b ). We were pleased to observe that all the natural products inhibited MurX to varying degrees in this assay (9–100% MurX inhibition at 200 nM, Supplementary Tables 3–5 ). Importantly, the most potent analogues against Mtb growth were also the most active MurX inhibitors in this screen ( Supplementary Figs 38 and 39 ). In a recent report by Ishizaki et al ., CPZEN-45, an analogue of the caprazamycin family of nucleoside antibiotics was shown not to inhibit MurX in M. smegmatis , but rather inhibited WecA, an enzyme involved in arabinogalactan biosynthesis in mycobacteria [40] . WecA also uses UDP-GlcNAc as a substrate but, unlike MurX, does not utilize Park’s nucleotide. As such, we also assessed inhibition of WecA by the sansanmycin analogues in our assay [40] . Interestingly, we did not observe inhibition of WecA by any of the compounds and, as such, the natural product analogues appear to be selective inhibitors of lipid I formation in peptidoglycan biosynthesis. 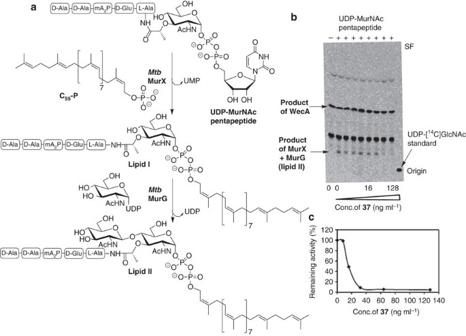Figure 4: Inhibition studies of the synthetic sansanmycin analogues againstMtbMurX. (a) Reactions catalysed byMtbMurX to generate lipid I andMtbMurG to generate lipid II. (b) Exemplar TLC assay fromMtbmc26230 membranes for the inhibition ofMtbMurX–MurG by dihydrosansanmycin analogue37(IC50=41 nM). Positive control=pacidamycin D19and tunicamycin. Ala, alanine; Glu, glutamate; mA2P,meso-diaminopimelic acid. Product of MurX=decaprenyldiphosphoryl-MurNAc-pentapeptide (lipid I), product of MurG=decaprenyldiphosphoryl-MurNAc-pentapeptide-GlcNAc (lipid II), product of WecA=decaprenyldiphosphoryl-GlcNAc. (c) Inhibition assay ofMtbMurX with dihydrosansanmycin analogue37(IC50=16 nM) using dansylated UDP-MurNAc pentapeptide as substrate.Km(app) UDP-MurNAc-pentapeptide=51±4 μM andVmax(app)=69±1.9 μM min−1;Km(app) polyisoprenylphosphate=56±9 μg ml−1(Supplementary Figs 40 and 41). Positive control tunicamycin: IC50=189 nM (Supplementary Fig. 46). Figure 4: Inhibition studies of the synthetic sansanmycin analogues against Mtb MurX. ( a ) Reactions catalysed by Mtb MurX to generate lipid I and Mtb MurG to generate lipid II. ( b ) Exemplar TLC assay from Mtb mc 2 6230 membranes for the inhibition of Mtb MurX–MurG by dihydrosansanmycin analogue 37 (IC 50 =41 nM). Positive control=pacidamycin D [19] and tunicamycin. Ala, alanine; Glu, glutamate; mA 2 P, meso -diaminopimelic acid. Product of MurX=decaprenyldiphosphoryl-MurNAc-pentapeptide (lipid I), product of MurG=decaprenyldiphosphoryl-MurNAc-pentapeptide-GlcNAc (lipid II), product of WecA=decaprenyldiphosphoryl-GlcNAc. ( c ) Inhibition assay of Mtb MurX with dihydrosansanmycin analogue 37 (IC 50 =16 nM) using dansylated UDP-MurNAc pentapeptide as substrate. K m(app) UDP-MurNAc-pentapeptide =51±4 μM and V max(app) =69±1.9 μM min −1 ; K m(app) polyisoprenylphosphate =56±9 μg ml −1 ( Supplementary Figs 40 and 41 ). Positive control tunicamycin: IC 50 =189 nM ( Supplementary Fig. 46 ). Full size image Having established inhibition of Mtb MurX by the dihydrosansanmycins at a single concentration, we next focused on three analogues which showed the most potent inhibition of Mtb and Mtb MurX in vitro (compounds 25 , 36 and 37 ). The TLC-based assay developed above was employed using a range of concentrations of a given analogue and IC 50 values of 54, 48 and 41 nM were determined for 25 , 36 and 37 , respectively (see Fig. 4b for assay plate for compound 37 ). Importantly, there was significant correlation between the IC 50 against Mtb MurX and the activity against Mtb H37Rv in vitro . To unequivocally determine that our lead sansanmycin analogues were inhibiting Mtb MurX exclusively (and not a combination of MurX and MurG), we established a complementary fluorescence-enhancement assay which measured the incorporation of an N -dansylated UDP-MurNAc pentapeptide (dansylated on the diaminopimelic acid moiety) using a modification to an assay reported for the E. coli orthologue by Bugg and co-workers [42] . Briefly, Mtb mc 2 6230 membranes were incubated with one of the lead analogues (compounds 25 , 36 or 37 ) and the N -dansylated UDP-MurNAc pentapeptide substrate and formation of lipid I monitored by excitation at 340 nm and detection at 530 nm. Gratifyingly, the fluorescence assay of 25 (IC 50 =30 nM), 36 (IC 50 =14 nM) or 37 (IC 50 =16 nM) demonstrated similar inhibitory potencies to those determined via the radiochemical assay. Importantly, these data verify that the compounds are selective inhibitors of Mtb MurX and that this is likely the mechanism of anti-mycobacterial activity. Furthermore, the development of this fluorescence assay now provides a higher throughput means to screen future Mtb MurX inhibitors. Intracellular anti-mycobacterial activity of lead analogues Having established that the three lead analogues were potent inhibitors of Mtb MurX, they were next assessed for their anti-mycobacterial activity in an intracellular assay. Specifically, THP-1 macrophages were infected with Mtb and the inhibition of mycobacterial growth measured in the presence of a range of concentrations of 25 , 36 or 37 . Gratifyingly, all of the natural product analogues maintained anti-mycobacterial activity intracellularly with IC 50 s of 1.57, 4.33 and 0.11 μM for 25 , 36 and 37 , respectively ( Supplementary Figs 31–33 ). This data provides encouragement that these compounds may serve as bonafide leads for future TB drug discovery efforts. Stability studies We finally assessed the stability of 25 , 36 and 37 in mouse and human plasma and mouse and human liver microsomes with each of the compounds showing excellent stability, with degradation half-lives of >7 h for human and mouse plasma and >160 min for human and mouse liver microsomes ( Supplementary Tables 6 and 7 ). Based on the potent inhibition of Mtb (both in vitro and intracellularly) and the promising stability data, these compounds now serve as exciting leads for the development of a further generation of sansanmycin derivatives with a view to developing a TB drug lead which operates through the inhibition of lipid I synthesis in Mtb. In summary, we have described the development of a robust divergent solid-phase synthetic strategy to rapidly access a library of dihydrosansanmycin natural product analogues. A number of potent inhibitors of Mtb were elucidated that possess activity both in vitro and in macrophages infected with the organism. The compounds were shown to potently inhibit the enzyme MurX, responsible for lipid I synthesis, a key intermediate en route to peptidoglycan in Mtb . Despite this mechanism of action, the natural product analogues possess selective activity against Mtb , with little to no activity against other pathogenic bacteria that also synthesize peptidoglycan. This selectivity provides a practical advantage for the potential use of these compounds as TB drugs as well as MurX as a TB drug target. Future work in our laboratories will focus on understanding the mechanism of this selectivity. Finally, the compounds were stable in plasma and against the action of liver microsomes which, together with the potent and selective activity against Mtb , lays the foundation for the development of TB drug leads based around this natural product scaffold in the future. Synthesis of sansanmycin analogues For materials, methods and complete details of synthetic procedures, see Supplementary Methods . 1 H, 13 C and 2D NMR spectra of compounds described in this manuscript can be found as Supplementary Figs 47–148 . In vitro inhibition assays Mtb Mtb H37Rv (ATCC 27294) was grown in Middlebrook 7H9 broth medium supplemented with OADC (Difco Laboratories, Detroit, MI, USA), 0.05% glycerol and 0.05% Tween-80. Freshly seeded cultures were grown at 37 °C, for ∼ 14 days, to mid-exponential phase (OD 600 0.4–0.8) for use in the inhibition assays. The effect of dihydrosansanmycin analogues against the growth of Mtb H37Rv was measured by a resazurin reduction microplate assay, using the procedure previously described by Taneja and Tyagi [34] . Mtb grown to mid-exponential phase (OD 600 0.4–0.8) was diluted to OD 600 0.002 in 7H9S medium (Middlebrook 7H9 with 10% albumin, dextrose, catalase (ADC, Moregate Biotech), 0.05% glycerol, 0.05% Tween-80, 1% tryptone; 96-well microtiter plates were set up with 100 μl inhibitors, serially diluted into 7H9S. Diluted Mtb (100 μl, representing ∼ 2 × 10 4 CFU ml −1 ) was added to each well. Plates were incubated for 5 days at 37 °C in a humidified incubator before the addition of a 0.02% resazurin solution (30 μl) and 20% Tween-80 (12.5 μl) to each well. Sample fluorescence was measured after 24 h on a BMG Labtech Polarstar Omega instrument with an excitation wavelength of 530 nm and emission at 590 nm. Changes in fluorescence relative to positive control wells ( Mtb H37Rv with no inhibitor) minus negative control wells (no Mtb H37Rv) were plotted for determination of MIC 50 values. Rifampicin (R3501) and isoniazid (I3377) were purchased from Sigma-Aldrich. Mtb inhibition using infected macrophage culture Mtb H37Ra strain (ATCC 25177) was grown in Middlebrook 7H9 broth medium supplemented with OADC (Difco Laboratories), 0.05% glycerol and 0.05% Tween-80. Freshly seeded cultures were grown at 37 °C, for ∼ 14 days, to mid-exponential phase (OD 600 0.4–0.8) for use in the inhibition assays and used to infect a human macrophage-like cell line (THP-1; ATCC TIB-202). THP-1 stocks were maintained at a culture density between 1 × 10 5 and 1 × 10 6 cells ml −1 in RPMI-1640 medium (with phenol red, 25 mM HEPES and 2 mM L -glutamine) supplemented with 10% FBS (FBS-500) and 0.05 mM β-mercaptoethanol. THP-1 cells were plated in 96-well tissue culture plates (Costar 3903; Corning) at a density of 1 × 10 5 cells/well with phorbol myristic acetate (PMA; 100 nM) added. THP-1 cells were left to differentiate for 48 h at 37 °C at 5% CO 2 . A cell suspension of sonicated Mtb H37Ra in RPMI-1640 cell culture medium was used to infect differentiated THP-1 cells at a multiplicity of infection of 5 for 4 h at 37 °C at 5% CO 2 . Supernatant was then removed from all wells, THP-1 cells were washed with 200 μl phosphate buffered saline (PBS) three times and were subsequently replenished with fresh RPMI-1640 cell culture medium and incubated for a further 24 h at 37 °C and 5% CO 2 . The sansanmycin analogues were diluted in fresh RPMI-1640 cell culture medium and added to corresponding wells. Positive controls were dissolved in 100% dimethyl sulfoxide (DMSO) and diluted in 7H9 broth (Difco Becton Dickinson) with 10% ADC, 0.05% glycerol and 0.05% Tween 80 before adding to the wells. After 72 h of incubation at 37 °C at 5% CO 2 , tissue culture medium containing the test compound was removed from the wells; the cells were washed with 200 μl PBS, and then lysed with sterile water containing 0.1% Triton X. Cell lysates were serially diluted, 1:10, and plated on Middlebrook 7H11/OADC (283010; Difco) agar through to 1:10,000 dilution. Agar plates were then incubated at 37 °C for 3–4 weeks, after which the bacteria colonies were counted and CFU ml −1 of cell lysates were determined. Screen against a panel of bacterial strains The effect of dihydrosansanmycin analogues against 15 clinically relevant Gram-positive and Gram-negative bacteria strains was evaluated using a procedure by Wong et al . [35] . Specifically, the screening panel consisted of six Gram-positive strains (BSL1: Bacillus subtilis 168, Staphylococcus epidermidis [ATCC 14990], Enterococcus faecium [ATCC 6569], Listeria ivanovii [BAA-139]); BSL2: S. aureus [ATCC 29213], methicillin-resistant S. aureus (MRSA) [BAA-44]) and nine Gram-negative strains (BSL1: Escherichia coli K12 [BW 25113], Acinetobacter baumanii [NCIMB 12457], Enterobacter aerogenes [ATCC 35029], Ochrobactrum anthropi [ATCC 49687], Providencia alcalifaciens [ATCC 9886]; BSL2: Yersinia pseudotuberculosis [IP2666 pIBI], Pseudomonas aeruginosa [ATCC 27835], Salmonella typhimurium LT2, Vibrio cholerae O1 [biotype El Tor A1552]). All staphylococcal strains, L. ivanovii and E. faecium were cultured in 10 ml of tryptic soy broth (17 g tryptone, 3 g soytone, 2.5 g dextrose, 5 g NaCl and 2.5 g dipotassium phosphate in 1 l distilled water; pH 7.5). P. alcalifaciens , O. anthropi , E. aerogenes and A. baumanii were grown in nutrient broth (Difco, USA), while B. subtilis , E. coli , V. cholerae , S. typhimurium , P. aeruginosa and Y. pseudotuberculosis cultures were grown in Luria Broth (10 g tryptone, 5 g yeast extract and 10 g NaCl in 1 l distilled water; pH 7.5). All three media were autoclaved at 121 °C for 30 min. Inoculated cultures were grown overnight in a shaker (200 r.p.m. ; 30 °C). Overnight saturated cell cultures of pathogenic strains were diluted 1:1,000 with fresh media and 30 μl of culture dispensed into each well of sterile clear 384-well plates. A total of 300 nl of DMSO prefraction stock solutions were pinned into screening plates using a Perkin Elmer Janus MDT robot. After inoculation, screening plates were stacked in a plate reader/shaker (Perkin Elmer EnVision) and OD 600 readings taken once per hour for 24 h. Computer generated growth curves for serially diluted pure compounds (with the top final screening concentration of 100 μM) were used to determine MIC values by correlating the OD 600 reading at the pre-exponential phase of the bacteria to the concentrations in individual wells. MurX enzyme inhibition assays Materials: UDP- N -acetyl- D -glucosamine [glucosamine- 14 C(U)] ([ 14 C]UDP-GlcNAc, Specific activity 300 mCi/mmol) was obtained from American Radio Chemicals, UDP-MurNAc-pentapeptide was obtained from BacWAN, University of Warwick, Coventry, UK ( www.warwick.ac.uk/bacwan ). Dansyl-labelled UDP-MurNAc-pentapeptide was synthesized from UDP-MurNAc-pentapeptide as described below. TLC Silica gel 60 F 254 plates were procured from Merck (Germany). All other chemicals used were at least analytical grade and were obtained from Sigma-Aldrich. Mtb mc 2 6230 was a generous gift from Dr William Jacobs, Albert Einstein College of Medicine, New York. Membrane preparation from Mtb mc 2 6230 Mtb mc 2 6230 was grown in 7H9 medium (supplemented with 0.5% (v/v) oleic acid, 0.5% (w/v) albumin, 0.2% (w/v) dextrose, 24 μg ml −1 D -pantothenate and 0.2% casamino acids). Washed cells were resuspended in Buffer A (50 mM MOPS pH 7.9, 5 mM MgCl 2 , 5 mM DTT, 10% glycerol (v/v)), at 2 ml g −1 of cells, and disrupted by probe sonication on ice with a Sanyo Soniprep 150 (10 cycles of 60 s on and 90 s off). The whole cell lysates were centrifuged at 5,000 g for 20 min at 4 °C. The supernatant was further centrifuged at 100,000 g (for 1 h at 4 °C) in an Optima TLX Ultracentrifuge (Beckman). The membrane-enriched pellets were washed in Buffer A followed by ultracentrifugation at 100,000 g . The washed pellets were resuspended in Buffer A, divided into aliquots and frozen at −80 °C. The protein concentration of the membrane-enriched fraction was estimated using a BCA protein assay kit (Pierce). Preparation of dansylated UDP-MurNAc pentapeptide Synthesis and purification UDP-MurNAc-pentapeptide was achieved by chemoenzymatic recapitulation of the cytoplasmic synthetic pathway in vitro [43] . Desalted UDP-MurNAc-pentapeptide in sterile water was mixed with an equal volume of acetone and allowed to react overnight with a 42-fold molar ratio of dansyl chloride with stirring. The reaction was quenched with a 10-fold molar excess of Tris-Cl pH 9 to dansyl chloride before rotary evaporation to remove solvents. Dried products were resuspended in 1 ml sterile water and purified by size exclusion chromatography on a Superdex peptide 10/300 column (GE Healthcare) pre-equilibrated with 1.5 CV 0.1 M ammonium bicarbonate. Dansylated UDP-MurNAc-pentapeptide is the first peak to elute in this procedure with a characteristic absorbance at 340 and 280 nm. Fractions containing the required product were freeze dried 4 times and resuspended in a small volume of sterile water. Quantification and purity were confirmed by absorbance and mass spectrometry, respectively. Radiochemical Mtb MurX inhibition assay Assay mixtures (200 μl) contained 50 mM MOPS pH 7.9, 5 mM MgCl 2 , 5 mM DTT, 10% glycerol (v/v), 0.1% CHAPS, 100 μM ATP, 25 μM UDP-MurNAc-pentapeptide, 0.5 μM [ 14 C] UDP-GlcNAc, and varying concentrations of inhibitor (initial screening was carried out at a single concentration of 200 nM and the most potent compounds were screened at a range of concentrations to determine IC 50 values, Supplementary Figs 34–37 ). Reactions were initiated by the addition of 400–500 μg of Mtb mc 2 6230 membrane protein and incubated at 37 °C for 1 h. Reactions were stopped by the addition of 6 ml of chloroform/MeOH (2:1), followed by low speed centrifugation and the organic extract was moved to a second tube. Extracts were back washed twice [once with water (800 μl) and then with chloroform/MeOH/water (3:47:48)], evaporated to dryness under a nitrogen stream, and dissolved in chloroform/MeOH (2:1 v/v). An aliquot was subjected to liquid scintillation counting (LS 6500, Beckman Coulter); a second aliquot was subjected to TLC (Silica gel 60 F 254 ) developed in chloroform/MeOH/water/ammonium hydroxide (88:48:10:1). Distribution of radioactivity was detected by phosphorimaging (Typhoon TRIO, Amersham Biosciences) and quantified with ImageQuant TL v2005 software (Amersham Biosciences). IC 50 values were calculated by using GraFit Software (Version 5.0.13). Fluorescence-based Mtb MurX inhibition assay Continuous fluorescence MurX assays (100 μl in volume) were carried out in vitro at 25 °C in an assay buffer consisting of 83 mM Tris pH 7.5, 21 mM MgCl 2 , 6% glycerol, 0.1% TritonX-100, 15 μM dansylated UDP-MurNAc-pentapeptide, 40 μg ml −1 polyisoprenyl phosphate and varying concentrations of inhibitor [42] . Reactions were initiated by the addition of 60–70 μg of Mtb mc 2 6230 membrane protein and fluorescence was monitored at 340 and 530 nm for excitation and emission, respectively. Assays were carried out in duplicate and IC 50 values were calculated using GraFit Software (Version 5.0.13, Supplementary Figs 42–44 ). A further inhibition assay was carried out for analogue 37 at an increased concentration of polyisoprenylphosphate (160 μg ml −1 , Supplementary Fig. 45 ). Assays were also performed at a fixed concentration of UDP-MurNAc-pentapeptide (15 μM) and a range of exogenous polyisoprenylphosphate concentrations. This enabled the determination of the apparent K m and V max values with respect to the polyisoprenylphosphate substrate. The endogenous polyisoprenylphosphate concentration in the extracted membrane was calculated to be 0.28 μg mg −1 of membrane protein. Stability studies in human and mouse plasma Human blood from nonidentifiable volunteer donors was sourced from the Australian Red Cross Blood Service under a supply agreement approved by the Monash Human Research Ethics Committee. Mouse blood was collected in-house under tissue harvesting protocols approved by the Monash Institute of Pharmaceutical Sciences Animal Ethics Committee. Pooled human and Swiss outbred mouse plasma samples were thawed and spiked with test compound solutions prepared in DMSO/acetonitrile/water (20:40:40) to provide a final compound concentration of 1,000 ng ml −1 and final DMSO and acetonitrile concentrations of 0.2% and 0.4% (v/v), respectively. Plasma was vortex mixed and aliquots (50 μl) were transferred to fresh microcentrifuge tubes and incubated at 37 °C. At various time points over the 6 h incubation period, duplicate plasma samples were removed and immediately snap-frozen in dry ice. All samples were stored frozen at −80 °C until analysis by LC–MS. Samples were processed by protein precipitation using a two-fold excess of acetonitrile followed by centrifugation. Analysis of the supernate was conducted using a Waters (Milford, MA) Acquity UPLC coupled to a Waters Micromass Quattro Premier mass spectrometer operated in positive electrospray ionization mode with multiple reaction monitoring. The cone voltage was 45 V, collision energy was 30, 30 and 40 V for 25 , 36 and 37 , respectively, and m / z transitions were 782.30>126.06 ( 25 ), 826.32>170.16 ( 36 ) and 888.39>126.06 ( 37 ). Processed samples (3 μl) were injected onto a Supelco Ascentis Express RP Amide column (50 × 2.1 mm, 2.7 μm) and analytes eluted using a water/acetonitrile (each containing 0.05% formic acid) gradient over 4 min with a flow rate was 0.4 ml min −1 . Sample concentrations were quantitated by comparison to a calibration curve prepared in blank human or mouse plasma. Stability studies in human and mouse liver microsomes The metabolic stability was assessed by incubating each test compound (0.5 μM) in duplicate with human and mouse liver microsomes (XenoTech, Kansas City, KS) at 37 °C and 0.4 mg ml −1 microsomal protein. The metabolic reaction was initiated by the addition of an NADPH-regenerating system and quenched at various time points over a 60 min incubation period by the addition of acetonitrile containing diazepam as internal standard. Control samples (containing no NADPH) were included and quenched at 2, 30 and 60 min to monitor for potential degradation in the absence of cofactor. Samples were centrifuged and the supernatant analysed by LCMS. Analysis was conducted using a Waters Acquity UPLC coupled to a Waters Xevo G2 QTOF mass spectrometer operated in positive electrospray ionization MS E mode with a cone voltage of 30 V. Samples (5 μl) were injected onto an Ascentis Express Amide column (50 × 2.1 mm, 2.7 μm) and eluted using a water/acetonitrile (both containing 0.05% formic acid) gradient over 4 min at a flow rate of 0.4 ml min −1 . Degradation rate half-lives and in vitro intrinsic clearance values were determined from the first order degradation profiles. Data availability Data supporting the findings of this study are available within the article and its Supplementary Information files and from the corresponding author upon reasonable request. How to cite this article: Tran, A. T. et al . Sansanmycin natural product analogues as potent and selective anti-mycobacterials that inhibit lipid I biosynthesis. Nat. Commun. 8, 14414 doi: 10.1038/ncomms14414 (2017). Publisher’s note : Springer Nature remains neutral with regard to jurisdictional claims in published maps and institutional affiliations.